The pore of voltage-gated potassium ion channels is strained when closed Voltage-gated potassium channels form potassium-selective pores in cell membranes. They open or close in response to changes in the transmembrane potential and are essential for generating action potentials, and thus for the functioning of heart and brain. While a mechanism for how these channels close has been proposed, it is not clear what drives their opening. Here we use free energy molecular dynamics simulations to show that work must be done on the pore to reduce the kink in the pore-lining (S6) α-helices, thereby forming the helix bundle crossing and closing the channel. Strain is built up as the pore closes, which subsequently drives opening. We also determine the effect of mutating the PVPV motif that causes the kink in the S6 helix. Finally, an approximate upper limit on how far the S4 helix is displaced as the pore closes is estimated. Voltage-gated potassium (Kv) channels form potassium-selective pores in lipid bilayers and are activated by membrane depolarisation. They are involved in many important physiological functions, for example, in the generation of action potentials [1] . Kv channels are typically homotetramers, and the first four transmembrane α-helices (S1–S4) of each monomer form the voltage-sensing domain ( Fig. 1a ). This is connected by the S4–S5 linker helix to the remaining two α-helices (S5 and S6); these come together with those of the other three monomers to form the central pore domain through which potassium ions and water molecules diffuse. The narrowest part of the pore, the selectivity filter [2] , is found towards the extracellular side of the protein ( Fig. 1b ). Immediately below the selectivity filter is a water-filled cavity approximately at the centre of the bilayer. In the closed structures of other K channels, the four helices equivalent to S6 (the TM2 or inner helices) are approximately straight, thereby forming a constriction point where the helices cross one another. In the two mammalian Kv channel structures [3] , [4] , the S6 helices are kinked such that these channels are assumed to be open and conductive. This kink occurs just N-terminal to a conserved PXP motif [5] . Proline cannot act as a hydrogen bond donor and therefore disrupts the backbone hydrogen bonding, leading to the kink. 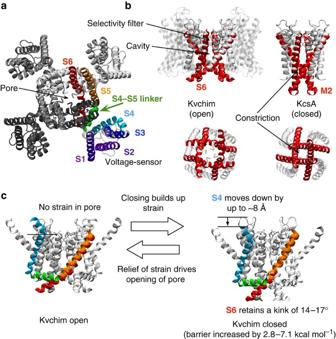Figure 1: Kv channels contain a central pore domain and four peripheral voltage-sensing domains. (a) Extracellular view of the tetrameric Kv1.2/2.1 paddle chimaera (Kvchim)4. The helices of one monomer are coloured and labelled. (b) Membrane and intracellular views of Kvchim (open) and KcsA (closed)2, respectively. The pore domains are coloured white and the inner helices are coloured red. (c) Schematic illustration of how the channel closes and opens with the average motions suggested by our simulations labelled. Figure 1: Kv channels contain a central pore domain and four peripheral voltage-sensing domains. ( a ) Extracellular view of the tetrameric Kv1.2/2.1 paddle chimaera (Kvchim) [4] . The helices of one monomer are coloured and labelled. ( b ) Membrane and intracellular views of Kvchim (open) and KcsA (closed) [2] , respectively. The pore domains are coloured white and the inner helices are coloured red. ( c ) Schematic illustration of how the channel closes and opens with the average motions suggested by our simulations labelled. Full size image It was first suggested by Woolfson et al . [6] that kinks introduced by prolines could help gate Kv channels. Subsequent molecular dynamics simulations [7] , [8] , [9] , [10] , [11] , [12] and accessibility [13] , [14] and mutagenesis [15] , [16] experiments supported and refined this hypothesis until it was confirmed by structural studies [3] , [4] . Long et al . [17] developed it further by proposing that when the transmembrane (TM) potential becomes negative, the voltage sensors are driven down in the membrane causing the S4–S5 linkers to press on the outside of the S6 helices straightening them, forming the constriction point ( Fig. 1c ). There are, however, two fundamental issues unaddressed by this description: while it explains how Kv channels close, it does not explain the origin of the physical forces that drive their opening. Secondly, it does not tell us how far the S4 helix, and hence the voltage sensor, must move to gate the pore. In this paper, we calculate how the free energy of the pore changes as the ends of the S6 helices are moved in the plane of the bilayer, much like the iris diaphragm of a camera. This reveals that work must be done on the central pore domain to straighten the S6 helices and close the channel. The pore is therefore strained when closed and the unwinding of this strain energy could drive the opening of the pore, thereby explaining how Kv channels open. Our results imply that, when the pore is closed, the S4–S5 linkers must remain in physical contact with the outside of the S6 helices. This places an indirect constraint on the motion of the S4 helices and will allow us to propose an approximate upper limit on how much the S4 helix moves as the pore closes. The voltage sensor must do work to straighten the S6 helices We assume that the central pore and the voltage sensors function as independent domains and that they communicate with one another primarily via the S4–S5 linker helix. Several independent lines of evidence support this assumption. Not only are the voltage sensors only peripherally connected to the pore domain ( Fig. 1a ), but it has also proved possible to resolve the structure of a single voltage sensor isolated from a whole channel [18] . Chimeric and mutagenesis experiments have demonstrated that different pore domains can be spliced into a Kv channel, provided the interface between the S4–S5 linker and the S6 helix is conserved [19] , [20] . Finally, membrane proteins homologous to the voltage sensor of Kv channels but without a pore domain have been found, further suggesting that voltage sensors can act as independent domains [21] , [22] . The basic residues that sense changes in voltage are confined to the S4 helix in the voltage sensor [23] , [24] , and therefore the electric field will only do work on the voltage sensors. If we combine this observation with our assumption, we recover the current mechanism as proposed by Long et al . [17] , where the voltage sensors (and therefore the electric field) influence the conformation of the central pore domain indirectly through movement of the S4–S5 linker helices. These are pivoted downwards by the voltage sensors as the transmembrane potential becomes negative, press on the outside of the S6 helices and close the channel [17] . We shall therefore study the energetics of the isolated pore domain of the Kv1.2/2.1 paddle chimaera (Kvchim) [4] —we shall refer to this as Kv1.2 CH —and infer how the energetics of the whole channel changes as the pore closes. After a careful series of equilibration simulations ( Supplementary Figure S1 ), we used free energy molecular dynamics methods to systematically move the ends of the S6 helices in the plane of the bilayer ( Fig. 2a ) while recording the mechanical response of the pore. As kinetic modelling suggests that the final step in closing the pore is cooperative [25] , biasing forces were applied in a concerted manner to move the ends of all four S6 helices simultaneously, like the iris diaphragm of a camera ( Fig. 2c ). We assumed that the data from each of the S6 helices were independent ( Supplementary Figures S2 and S3 )—this allowed us to combine the data. We investigated the convergence of this data set and estimated a correlation time ( Supplementary Figure S4 ), permitting us to calculate a single converged two-dimensional (2D) potential of mean force (PMF) map ( Fig. 2 ). This has a single broad minimum. The coordinates of the S6 helices from both mammalian Kv structures [3] , [4] lie 1.2 kcal mol −1 above the bottom of the well. The statistical error is estimated to be <0.2 kcal mol −1 ( Supplementary Figure S4 ) over most of the region sampled. To independently check this result, we ran unbiased simulations of KcsA with a mutated M2 helix. Introducing the PVPV motif into KcsA led to kinks rapidly forming whereas the M2 helices remained approximately straight in the wild-type channel ( Supplementary Figure S5 ), consistent with this motif destabilising the closed state. 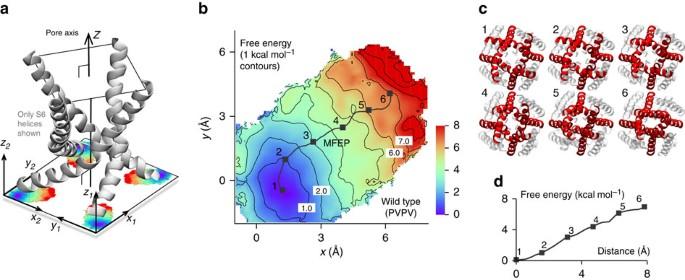Figure 2: The S6 helices of Kv1.2CHprefer to remain kinked. (a) Schematic showing the extent of the motion of the S6 helices and how the S6 and pore coordinate systems are defined. The origin of each S6 coordinate system is defined as the position of the S6 helix in the Kvchim structure4. (b) The final converged (Supplementary Figure S4) 2D potential of mean force (PMF) showing how the free energy varies as the ends of the S6 helices of Kv1.2CHare moved in the (x–y) plane of the membrane. The positions of the equivalent residues in the structures of Kv1.2 (ref.3), closed KcsA (ref.2) and MlotiK1 (ref.60) are also plotted. The minimum free energy path (MFEP) between the centre of the well and the coordinates for KcsA is drawn. Six reference points are labelled; these are referred to in other panels of this figure as well as in other figures. Contours are drawn every 1 kcal mol−1. (c) The conformation of the S6 helices (in red) when viewed intracellularly are shown. (d) The free energy increases along the MFEP, requiring 7.0 kcal mol−1per monomer to straighten the helices to the same extent as KcsA. The estimated errors are smaller than the filled squares and so are not plotted. Figure 2: The S6 helices of Kv1.2 CH prefer to remain kinked. ( a ) Schematic showing the extent of the motion of the S6 helices and how the S6 and pore coordinate systems are defined. The origin of each S6 coordinate system is defined as the position of the S6 helix in the Kvchim structure [4] . ( b ) The final converged ( Supplementary Figure S4 ) 2D potential of mean force (PMF) showing how the free energy varies as the ends of the S6 helices of Kv1.2 CH are moved in the ( x–y ) plane of the membrane. The positions of the equivalent residues in the structures of Kv1.2 (ref. 3 ), closed KcsA (ref. 2 ) and MlotiK1 (ref. 60 ) are also plotted. The minimum free energy path (MFEP) between the centre of the well and the coordinates for KcsA is drawn. Six reference points are labelled; these are referred to in other panels of this figure as well as in other figures. Contours are drawn every 1 kcal mol −1 . ( c ) The conformation of the S6 helices (in red) when viewed intracellularly are shown. ( d ) The free energy increases along the MFEP, requiring 7.0 kcal mol −1 per monomer to straighten the helices to the same extent as KcsA. The estimated errors are smaller than the filled squares and so are not plotted. Full size image As there is no structure of a closed Kv channel, we initially assumed that the S6 helices of Kv1.2 CH resemble the M2 helices of KcsA [2] (that is, are approximately straight) when the pore is closed. Previous studies have also made this assumption [12] , [26] , [27] . We calculated the minimum free energy path (MFEP) across the 2D PMF between the points representing the conformations of the pore-lining helices of Kvchim (open) and KcsA (closed) using the nudged elastic band method [28] . The free energy increases along the MFEP ( Fig. 2b ), reaching 7.0 kcal mol −1 per monomer at the end. Along the MFEP, the error is estimated to be <0.2 kcal/mol ( Supplementary Figure S4 ), and the average kink angle of the S6 helices decreases from 26° to 12° ( Supplementary Figure S6 ). We conclude that the pore domain has a higher energy when it is closed, hence we describe the pore as strained. The voltage sensors must therefore do work on the pore domain to straighten the S6 helices and close the pore. As the 2D PMF is approximately flat perpendicular to the MFEP, other closing paths are also probable. This explains why we occasionally observe the symmetry of the pore breaking from four- to two-fold ( Supplementary Figure S7 ), an effect seen in other simulations of Kv channels [29] . The S6 helices need not straighten fully to close the pore To test our assumption that the S6 helices of Kv1.2 CH are as straight as the M2 helices of KcsA when the pore is closed, we determined when along the MFEP the pore becomes impermeable to a potassium ion. This was done by calculating the one-dimensional (1D) PMF of moving a potassium ion from below the channel, past the constriction point, and into the central cavity. Water is present, so this approach naturally includes any energetic cost of dehydrating the cation. Fifteen 1D PMFs were calculated covering a range of pore radii and, as expected, the height of the energetic barrier faced by a potassium ion increases as the average pore radius decreases ( Fig. 3a and Supplementary Figures S8 and S9 ). This is well fitted by an exponential—a theoretical study that analysed the permeation of water through simple hydrophobic model pores found a similar relationship [30] . Using this function, we predicted how the height of the energetic barrier to ion permeation changes along the MFEP ( Fig. 3b and Supplementary Figure S9 ). 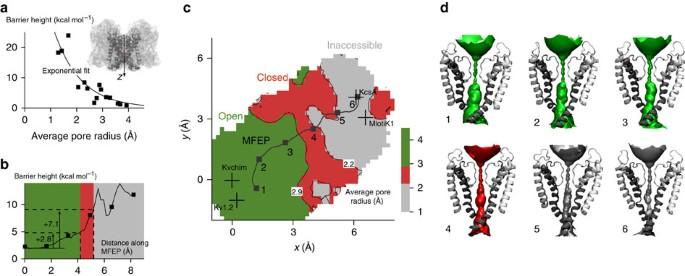Figure 3: The S6 helices remain kinked when the pore is closed. (a) The height of energetic barrier faced by a potassium ion is extracted from a series of fifteen 1D potential of mean forces (PMF) (Supplementary Figure S8) and then plotted against the average pore radius. The relationship is well fitted by an exponential and shows that as the pore radius decreases, the free energy required to move a potassium ion past the constriction point increases. (b) Using this relationship, the height of the energetic barrier is predicted along the minimum free energy path (MFEP). The channel is empirically defined as open (green) where the barrier is <2.7 kcal mol−1, closed (red) where the barrier has been increased by between 2.8 and 7.1 kcal mol−1and inaccessible (grey) where the barrier has increased by >7.1 kcal mol. This colour scheme is used in the remaining panels. (c) The 2D PMF inFigure 2bcan be divided into open, closed and inaccessible regions. (d) To illustrate this, the accessible pore surfaces taken from six points along the MFEP are shown. For clarity, only two of the four monomers are drawn and the S6 helices are colored dark grey. Figure 3: The S6 helices remain kinked when the pore is closed. ( a ) The height of energetic barrier faced by a potassium ion is extracted from a series of fifteen 1D potential of mean forces (PMF) ( Supplementary Figure S8 ) and then plotted against the average pore radius. The relationship is well fitted by an exponential and shows that as the pore radius decreases, the free energy required to move a potassium ion past the constriction point increases. ( b ) Using this relationship, the height of the energetic barrier is predicted along the minimum free energy path (MFEP). The channel is empirically defined as open (green) where the barrier is <2.7 kcal mol −1 , closed (red) where the barrier has been increased by between 2.8 and 7.1 kcal mol −1 and inaccessible (grey) where the barrier has increased by >7.1 kcal mol. This colour scheme is used in the remaining panels. ( c ) The 2D PMF in Figure 2b can be divided into open, closed and inaccessible regions. ( d ) To illustrate this, the accessible pore surfaces taken from six points along the MFEP are shown. For clarity, only two of the four monomers are drawn and the S6 helices are colored dark grey. Full size image Single-channel patch clamp recordings can only detect falls in Shaker Kv channel conductances of ~100-fold [31] that is, down to a unitary conductance of ~0.2 pS. A single Shaker channel would therefore be classified as closed when the energetic barrier to ion permeation that forms at the constriction point has increased by at least 2.8 kcal mol −1 . Soler-Llavina et al . [31] estimated that at −100 mV, the conductivity of Shaker is reduced by at least 10 5 -fold, corresponding to an increase in the barrier of 7.1 kcal mol −1 . This is an upper limit on the height of the energetic barrier, as the TM potential in mammalian cells is rarely more negative than −100 mV. Kvchim has been shown to be electrophysiologically similar to Shaker [32] , so we shall operationally define it to be closed when the energetic barrier to ion permeation at the constriction point has increased by a value in the range of 2.8–7.1 kcal mol −1 . Kv1.2 CH is therefore open for around the first half (51%) of the MFEP, closed in the following small region (51–64%) and does not sample the remainder of the MFEP ( Fig. 3 ). The voltage sensors must therefore do 3.5–4.5 kcal mol −1 of work on each S6 helix to operationally close the pore. Using a simple elastic model Choe and Grabe [11] estimated that two straight conformations of the S6 helix were 2.5–3.8 kcal mol −1 per monomer higher in energy than the observed kinked conformation, consistent with our result. The average kink angles of the S6 helices corresponding to the open, closed and inaccessible regions defined above are 26–18°, 17–14° and 13–12°, respectively ( Supplementary Figure S6 ). The S6 helices therefore retain a significant kink, even when the pore is closed, as proposed by del Camino et al [14] . To independently validate the conformations of the pore, we rolled probes of varying radii over the S6 helices and estimated the change in accessibility as the pore becomes closed. We found that residues 403 and 407 are more accessible when the pore is open ( Supplementary Figure S10 ), in agreement with cysteine accessibility experiments [13] . As a proline at the ( i )th position cannot form a backbone hydrogen bond with the amino acid at the ( i −4)th position, one would expect the prolines in the PXP motif to affect the dihedral angles of the residues a turn earlier (Thr397 and Ala399). Analysing the average backbone dihedral angles shows that only the φ angles of Pro401 and Leu400 and the ψ angle of Pro401 ( Supplementary Figures S11 and S12 ) change significantly along the MFEP. The effect of the PVPV motif on the dihedral angles of the S6 helical bundle is hence more complex than we might expect. The PVAV S6 helices are predicted to be less kinked Next, we investigated the effect of mutating the second proline in the PVPV motif to alanine (P403A). The PVAV mutant is known to conduct but the voltage-activation curve is shifted to more positive voltages and the channel opens more slowly [16] , [33] . The 2D PMF again has a single minimum, but its centre is shifted towards the coordinates of the M2 helices of KcsA ( Fig. 4 and Supplementary Figure S13 ). Our simulations therefore predict that the PVAV S6 helices are less kinked than the wild-type, consistent with the stabilisation of the closed state seen in the experiment [33] . This result also give us additional confidence that the 2D PMF for the wild-type pore ( Fig. 2 ) is correct as it indicates that it is unlikely that the form of the 2D PMF is simply a result of the simulations distorting the initial structure, as this would only ever result in a minimum centred on the origin. 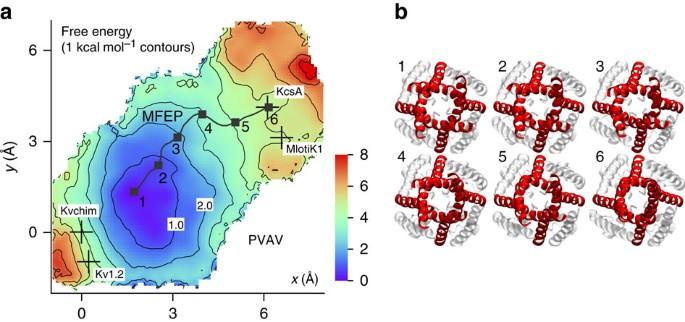Figure 4: The minimum in the PVAV mutant 2D potential of mean force (PMF) is shifted compared with wild-type. (a) The position of the minimum in the 2D PMF for the PVAV mutant Kv1.2CHis shifted towards KcsA compared with the wild type. As in the wild-type 2D PMF, the last 3 ns of each umbrella simulations is used. The positions of the equivalent residues in the structures of Kv1.2 (ref.3), closed KcsA (ref.2) and MlotiK1 (ref.60) are also plotted. Six reference points are labelled. Contours are drawn every 1 kcal mol−1. (b) The conformation of the S6 helices (in red) when viewed intracellularly. Figure 4: The minimum in the PVAV mutant 2D potential of mean force (PMF) is shifted compared with wild-type. ( a ) The position of the minimum in the 2D PMF for the PVAV mutant Kv1.2 CH is shifted towards KcsA compared with the wild type. As in the wild-type 2D PMF, the last 3 ns of each umbrella simulations is used. The positions of the equivalent residues in the structures of Kv1.2 (ref. 3 ), closed KcsA (ref. 2 ) and MlotiK1 (ref. 60 ) are also plotted. Six reference points are labelled. Contours are drawn every 1 kcal mol −1 . ( b ) The conformation of the S6 helices (in red) when viewed intracellularly. Full size image The S4 helix is displaced by up to ~8 Å when the pore closes Our results suggest that closing the pore of wild-type Kv1.2 CH requires work to be done which is derived from the electric field. The electric field exerts a force on the basic residues of the S4 helix, which drives them towards the intracellular side of the membrane, causing the S4–S5 linker helices to pivot, touch and then push on the outside of the S6 helices, reducing their kink angle and forcing the pore into a strained (high energy) state. We infer that the pore will only remain closed if a force is continuously applied by the S4–S5 linkers to the outside of the S6 helices—otherwise the pore would spring open to relieve the strain. When the pore is closed, the S4–S5 linkers must therefore remain in physical contact with the outside of the S6 helices. As the S4 helix is immediately N-terminal to the S4-S5 linker, this indirectly constrains the conformations the S4 helices can adopt in the membrane as the pore closes. To model this behaviour, the whole channel, including the voltage sensors and the T1 domain, was described using a combined elastic network and coarse-graining approach ( Supplementary Figure S14 ). When the channel is open, the S4–S5 linker rests on the outside of the S6 helix [3] , [4] . Chimeric studies have demonstrated that the interface between the linker and the S6 helix is optimised [19] and mutating residues at the interface also disrupts gating [20] . We have assumed that this interface is preserved throughout pore closure. This was enforced by adding extra elastic network restraints between the residues at the interface [20] , thereby ensuring that both the interface between the S6 helix and the S4–S5 linker and their relative orientation were maintained during the coarse-grained molecular dynamics simulations. The elastic network also prevented the S4 helix from changing its overall secondary structure, but otherwise, it was free to move up and down in the bilayer and rotate relative to the bilayer normal. Each simulation generates an ensemble of conformations the S4 helix can adopt in a lipid bilayer given that it is surrounded by the remainder of the voltage sensor, and we have enforced the constraint that the interface between the S4–S5 linker and the S6 helix is preserved. Repeating simulations using a range of pore conformations, each with a different pore radii, enabled us to estimate how the ensemble of conformations that S4 can adopt changes as the pore is closed, or equivalently as we traverse the MFEP. The simulations do not directly estimate how far the S4 helices must be displaced along the membrane normal to close the pore. This is, we presume, a subset of the possible S4 conformations that is sampled by the simulations. Determining the maximum displacement of the centre of mass towards the intracellular medium therefore yields an approximate upper limit on the possible motion of S4. As we traverse the MFEP, the centres of mass of the S4 helices are displaced by up to 10 Å ( Fig. 5 ), and S4 adopts angles with respect to the bilayer normal in the range of 10–60° ( Supplementary Figure S15 ). If we exclude from our analysis the region we earlier defined to be inaccessible, then the value for the maximum observed displacement drops to 8 Å. Our results suggest that the centre of mass of the S4 helix is displaced by up to ~8 Å towards the intracellular medium as the pore is closed. 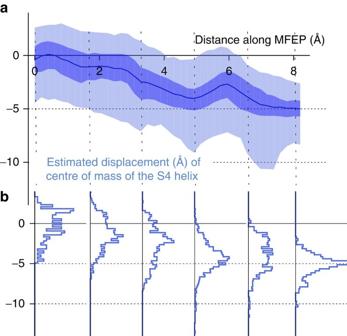Figure 5: The wild-type PVPV S4 helix is displaced vertically by up to ~8 Å when the pore is operationally closed. (a) The centre of mass of the S4 helix moves down towards the intracellular side of the lipid bilayer as the kink in the S6 helices is reduced, closing the pore. The average along the minimum free energy path is drawn as a blue line. The ranges 25–50% and 2–98% are shaded medium and light-blue, respectively. (b) The distributions are also plotted for six reference points. Figure 5: The wild-type PVPV S4 helix is displaced vertically by up to ~8 Å when the pore is operationally closed. ( a ) The centre of mass of the S4 helix moves down towards the intracellular side of the lipid bilayer as the kink in the S6 helices is reduced, closing the pore. The average along the minimum free energy path is drawn as a blue line. The ranges 25–50% and 2–98% are shaded medium and light-blue, respectively. ( b ) The distributions are also plotted for six reference points. Full size image The current explanation of how Kv channels gate is that as the transmembrane potential becomes negative, the voltage sensors are driven down in the bilayer, pulling on the N-terminal end of the S4–S5 linkers, causing them to pivot [17] . These helices then press on the outside of the S6 helices, reducing their kink angle and as a result an energy barrier to ion permeation grows at the helix bundle crossing until current can no longer be detected. This description does not identify the origin of the physical forces that cause the pore to subsequently open. Our results suggest that the electric field, via the voltage sensors, pushes the pore domain into a strained (high energy) state ( Fig. 2 ), as the channel becomes closed. We infer that (1) the kink created by the PVPV motif favours the open state, (2) the potential energy created while the pore closes is mainly stored in the S6 helices, as the structural changes of the pore are mainly confined to these helices ( Supplementary Figure S16) , and (3) the S6 helices of the wild-type paddle chimaera retain a kink even when closed, as suggested by del Camino et al . [14] Finally, we predict that the S6 helices of the PVAV mutant have less of a kink than the wild-type channel. We propose a model that explains how Kv channels open: as the transmembrane potential becomes positive, the voltage sensors move back up in the bilayer, causing the S4–S5 linkers to pivot upwards allowing the S6 helices to ‘spring back’ to their low energy kinked conformation ( Fig. 1c ). The opening of the pore is therefore driven by the relief of strain in the pore; the closing is instead driven by the downwards displacement of the voltage sensor brought about by the electric field. This asymmetry potentially explains the observed differences in both the off- and on-gating currents [34] and the activation kinetics, in particular, how mutating the S6 helices often affects the opening, but not the closing kinetics [33] . The strain in the pore is also likely to make it harder to crystallise a closed Kv channel unless the strain is reduced or removed, perhaps by mutation of the S6 helix. Our results suggest that each voltage sensor must do 3.5–4.5kcal mol −1 of work (14–18 kcal mol −1 per channel) to close the pore—that is, Kvchim without any voltage sensors attached (Kv1.2 CH ) would almost always be open. Chowdhury and Chanda [35] have recently calculated from electrophysiological measurements that at 0 V, the open state of Shaker is more stable than the closed state by 14.6 kcal mol −1 . This is in good agreement with our result, assuming that no energy is stored in or dissipated by the voltage sensors. Based on an extensive mutagenesis study of Shaker , Yifrach and MacKinnon [36] instead suggested that the pore is intrinsically more stable when closed, although they were unable to experimentally study either proline in the PVPV motif. Further work by Labro et al . [15] showed that mutating the prolines destabilised the open state, consistent with our result. In general, it is very difficult to dissect the thermodynamics of a voltage-gated ion channel. We have approached this by assuming that the pore domain and voltage sensors are independent, which allowed us to study the pore domain in isolation. This further assumes a tight coupling between the S4–S5 linkers and the S6 helices, which is not known, as the experimental evidence is mixed [37] , [38] . Detailed kinetic modelling can also isolate some of the thermodynamic steps in the gating of Kv channels. For example, the last activation step in the kinetic model proposed by Zagotta et al . [25] is the opening of the pore domain. By examining the temperature dependence of the gating of Shaker , Rodríguez et al . [39] were able to suggest by applying this kinetic model that, when the voltage sensors are activated, the closed pore is higher in energy by 1.6 kcal mol −1 , consistent with our result. Naturally, there are shortcomings in our approach. Our model that most of the energy derived from voltage sensor movement is stored in the pore domain may be oversimplistic. Some of the energy may be stored in the voltage sensors, as has been suggested for a sodium channel [40] . Our assumption that the voltage-sensing and pore domains are independent may also be an oversimplification. The voltage sensors may modulate the pore in more complex ways. For example, the ILT mutation within the Shaker voltage sensor is known to decouple most of the gating charge movement from channel opening [41] . Our model cannot explain this as it predicts that the pore would open as soon as the voltage sensors activate. The second issue with the current description of how Kv channels gate [17] is that it does not describe how the S4 helices move to cause pore closure. This remains disputed and a range of mechanisms have been proposed and subsequently refined (reviewed elsewhere [42] , [43] , [44] ). By building on our earlier results, we have been able to estimate that to close the pore, the centre of mass of the S4 helices is displaced towards the intracellular medium by up to ~8 Å. This is consistent with several [45] , [46] , [47] but not all [48] biophysical experiments. As indicated, this result is approximate, as our approach has several shortcomings. A coarse-grained model is generally less accurate than an atomistic model, and specifically does not permit changes in secondary structure (for example, the S4 helix cannot become a 3 10 helix). We have also assumed that the interface between the S4–S5 linker and S6 identified by the experiment of Labro et al . [20] is maintained throughout. Finally, the models rely on the earlier atomistic simulations, including the 2D PMF ( Fig. 2 ), and so are models built on models with the attendant conflation of errors. Our approach, however, is novel and is based on a purely mechanical and geometrical argument and so does not depend on the exact details of how the electric field is focussed. Our inference that when the pore is closed the S4–S5 linker must be physically contacting the outside of the S6 helix is not subject to these shortcomings, and so, could be used as a starting point for further experimental or theoretical estimates of the displacement of S4. Jensen et al . [29] , [49] have carried out very extensive unbiased molecular dynamics simulations of both Kv1.2 and Kvchim both with and without the voltage sensors under an applied electric field. They observe a dewetting process whereby water and ions leave the cavity and the S6 helices straighten, come together and close the channel. As a result, they conclude that the closed state is more stable: this disagrees with our main result ( Fig. 2 ). In their simulations, the S4 helices were displaced by ~15 Å, which is at the high end of the range of motions suggested by biophysical experiments [45] , [46] , [47] , [48] . This could possibly be due to the high magnitude of the applied electric field; more sophisticated methods for simulating the electrical field across a cell membrane are required if we are to accurately simulate the conduction and gating of Kv channels. Whatever the origins of these discrepancies, it is clear that more work, both experimental and theoretical, needs to be done before we can fully explain how voltage-gated ion channels open and close. Our proposed mechanism relies on the pore-lining helix possessing a kink due to a PXP motif. There must also exist other more general mechanisms that explain how ion channel pores open and close as they do not all possess such motifs. The dewetting observed by Jensen et al . [29] , [49] is one candidate. Simulation studies have also shown that glycines make α-helices more flexible [7] , [10] , and it has been suggested that a highly conserved glycine [5] present in the pore-lining helix of many potassium channels can form a hinge [50] . Adding prolines to the pore-lining helices of channels that lack them often has quite a dramatic effect, for example, this increases the open probability and mean burst duration of the GIRK4 channel [51] . In NaChBac introducing a proline leads to a channel that requires only a small change in TM voltage to open [52] . These results suggest that prolines introduce a bias towards open, and we assume, kinked conformations. Yet the glycine in Shaker , which has a PVPV motif, is required [36] , indicating it is also important, perhaps in permitting the conformational changes occurring lower down the helix ( Supplementary Figures S11 and S12 ). In summary, when the membrane potential repolarises, the S4 helices of Kvchim are displaced towards the intracellular medium by up to ~8 Å, causing the S4–S5 linkers to pivot, touch and push on the outside of the pore-lining S6 helices, straightening them (but not completely) and closing the pore. This requires each voltage sensor to do 3.5–4.5 kcal mol −1 of work, which is stored as an elastic strain energy in the central pore domain—hence, we describe the whole channel as frustrated when it is closed. We infer that it is the PXP motif in the S6 helix that introduces the kink and this favours the open state of the pore. Upon depolarisation, the voltage sensors move towards the extracellular side of the membrane, releasing the S6 helices that spring back to their low energy, kinked state, relieving the strain in the pore and opening the channel ( Fig. 1c ). Wild-type S6 2D PMF The voltage sensors of the paddle chimera were removed, leaving only the pore region (residues 321–417). A bilayer was added by allowing lipids to self-assemble around the protein using coarse-grained simulations [53] . The final structure was then converted back to an atomistic representation [54] . Water was added and K + ions were placed in the cavity of the channel and at the S4, S2 and S0 positions, with waters placed at the S1 and S3 positions. The cavity of the pore was filled with waters using voidoo and flood [55] . Finally, 12 sodium ions were added to make the simulation unit cell electrically neutral. We used the CHARMM27 forcefield with the CMAP correction and therefore all hydrogens are included and water is described using the TIP3P model. The simulation unit cell comprised 72,354 atoms, including 227 POPC lipids. The energy of the system was minimised using NAMD2.7, and then, the temperature was increased from 100 K to 300 K in 20 K steps, each running for 40 ps. The positions of the backbone atoms of the first turn of S6 (residues 380-383 incl.) were fixed and the positions of the heavy atoms of the lipid headgroups were constrained in the z direction ( k =10 kcal mol −1 Å −2 ). The constraints were then reduced 10-fold and a further 60 ps of MD was run at 310 K, before being removed. This and all subsequent simulations were run in the NpT ensemble. The pressure was maintained at 1 atm using a Berendsen barostat, which was applied anisotropically with a compressibility of 4.46 × 10 −5 bar −1 and a relaxation time of 0.2 ps. The temperature was maintained at 310 K by a Langevin thermostat with a damping coefficient of 1.0 ps −1 . SHAKE and SETTLE were applied to constrain the length of all bonds that involve a hydrogen, allowing an integration time step of 2 fs. Electrostatic forces were calculated using the particle mesh Ewald method with a grid spacing of 1 Å, and van der Waals forces were truncated at 12 Å with a switching function applied from 10 Å. The centre of mass of the heavy atoms of the last two turns of the S6 helices (residues 410–417 incl.) in the xy plane are recorded. The origin of this plane is defined by the paddle chimaera. Position constraints of 5 kcal mol −1 Å −2 were applied to the backbone atoms of the first turn of S6 (residues 380–383 incl.) throughout. The pore axis was therefore well-defined and the xy coordinates could be calculated using linear algebra. To prevent the S6 helices snapping the distances of the last three backbone hydrogen bonds of S6 were constrained by a half-harmonic potential with a spring constant of 10 kcal mol −1 Å −2 with an equilibrium separation of 2.8 Å. The TclForces module of NAMD was used, which allowed on-the-fly calculation of the positions of the last two turns of S6, the output of bespoke data files and application of the appropriate umbrella force. The system was equilibrated for 10 ns with the S6 helices held at the origin of the xy plane by a restraining force ( k =2 kcal mol −1 Å −2 ). Seven 5-ns simulations were then seeded, each at a different S6 coordinate ( Supplementary Figure S1 ), still with k held at 2 kcal mol −1 Å −2 . The magnitude of the biasing force was capped at 2 kcal mol −1 Å −1 for the first 1 ns. Only conformations of the pore that were roughly symmetrical and whose S6 helices remained helical were extracted and used as potential seeds for the next step. 80 × 1 ns umbrellas were then run. These were arranged trigonally with k =8.0 kcal mol −1 Å −2 . Again the magnitude of the biasing force was capped for the first 0.1 ns. A preliminary 2D PMF was then calculated using the weighted histogram analysis method [56] , and the MFEP was estimated using the nudged elastic band method [28] . The coordinates of the MFEP were used to define 20 new umbrella simulations. A further 37 beads were distributed around the MFEP. Each of these 57 umbrella simulations was run for 10 ns, as before. This process is illustrated in Supplementary Figure S1 . The 2D PMF required 0.7 μs of molecular dynamics simulations. Spring constants of either 5.0 or 8.0 kcal mol −1 Å −2 were assigned, again with the magnitude of the force capped for the first 50 ps. The 2D PMF was determined to be converged after 7 ns ( Supplementary Figure S4 ). All other analysis was done using VMD, HOLE or MDAnalysis [57] . Graphs were plotted using gnuplot and images rendered using VMD. Differences for the mutant S6 2D PMF The proline-to-alanine mutation was made using the mutator plugin of VMD. We kept the trigonal arrangement for the umbrella simulations throughout. This is more efficient and meant we only need to run 46 umbrella simulations for the PVPV mutant compared with 57 for the wild type. 1D potassium PMFs The Z coordinate of the potassium ion was defined relative to the selectivity filter [58] . Umbrella potentials were placed at 0.5 Å intervals covering the range −44.0≤ Z ≤−12.0 Å, making a total of 65 umbrella simulations for each 1D PMF. A spring constant of 10 kcal mol −1 Å −2 was used, and the magnitude of the applied force was capped for the first 50ps of each 250-ps simulation. A flat-bottomed cylindrical constraint was applied with a radius 8.0 Å and a spring constant of 10 kcal mol −1 Å −2 . Fifteen PMFs were calculated ( Supplementary Figure S8 ), each with the S6 helices restrained in different conformations. We estimated that the 1D PMFs were converged after 100 ps. Calculating all 15 × PMFs required 0.244 μs of molecular dynamics simulation. Coarse-grained simulations Voltage sensors and the tetramerisation (T1) domain were fitted back and added onto a series of idealised pore tetramers ( Supplementary Figure S14 ), such that the series sampled the whole of the MFEP. Each conformation was converted to a coarse-grained representation [59] , with elastic network model (ENM) bonds added between any two beads separated by <7 Å. ENM bonds between, for example, the voltage sensor and the pore were removed. Additional ENM bonds were added between residues forming the interface between the linker and the S5 helix [20] . The pore was made more rigid by adding bonds between any heavy bead separated by 9 Å, with a spring constant of 10,000 kJ mol −1 nm −2 . The resulting structure was fitted onto an already equilibrated coarse-grained self-assembly simulation of a wild-type paddle chimaera in a box of 374 POPC lipids. Any clashing waters and lipids were then removed resulting in, for example, 340 POPC lipids, 13,100 waters beads and 137 sodium and 97 chloride ion beads. Using GROMACS 4.5.3, the energy of the simulation unit cell was then minimised for 1,000 steps using the steepest descent method, followed by 1 ns of molecular dynamics. Then, 100 ns of molecular dynamics were run. Conventional coarse-grained run parameters were used [53] . These simulations generated 15 μs of molecular dynamics. How to cite this article: Fowler, P. W. et al . The pore of voltage-gated potassium ion channels is strained when closed. Nat. Commun. 4:1872 doi: 10.1038/ncomms2858 (2013).